Variant calling from scRNA-seq data allows the assessment of cellular identity in patient-derived cell lines 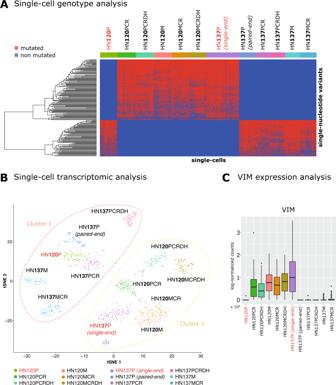Fig. 1: Analysis of single-cell mutational and gene expression profiles of patient-derived OSCC cell lines from scRNA-seq data. AThe heatmap including the mutational profiles of all single cells of the HN120 and HN137 datasets is displayed (-P: primary line, -M: metastatic line, -CR: after cisplatin treatment, -CRDH: after drug-holiday). Red entries mark cells displaying a given SNV. For the ID of single cells and SNVs please refer to Supplementary Data1and2.BThe t-SNE plot generated from the gene expression profiles of all single cells for all datasets is shown (see the SI for additional details).CThe distribution of the expression level ofVIMon all single cells is shown with boxplots for all datasets. Further information on research design is available in the Nature Research Reporting Summary linked to this article.